Clusterin and LRP2 are critical components of the hypothalamic feeding regulatory pathway Hypothalamic feeding circuits are essential for the maintenance of energy balance. There have been intensive efforts to discover new biological molecules involved in these pathways. Here we report that central administration of clusterin, also called apolipoprotein J, causes anorexia, weight loss and activation of hypothalamic signal transduction-activated transcript-3 in mice. In contrast, inhibition of hypothalamic clusterin action results in increased food intake and body weight, leading to adiposity. These effects are likely mediated through the mutual actions of the low-density lipoprotein receptor-related protein-2, a potential receptor for clusterin, and the long-form leptin receptor. In response to clusterin, the low-density lipoprotein receptor-related protein-2 binding to long-form leptin receptor is greatly enhanced in cultured neuronal cells. Furthermore, long-form leptin receptor deficiency or hypothalamic low-density lipoprotein receptor-related protein-2 suppression in mice leads to impaired hypothalamic clusterin signalling and actions. Our study identifies the hypothalamic clusterin–low-density lipoprotein receptor-related protein-2 axis as a novel anorexigenic signalling pathway that is tightly coupled with long-form leptin receptor-mediated signalling. Obesity has become one of the most common metabolic disorders worldwide [1] . Obesity results from chronic excess energy intake over energy expenditure. The hypothalamus, located at the base of brain, has a key role in the physiologic regulation of energy intake and expenditure [2] . An important component of this regulation is the ability of the hypothalamus to sense metabolic signals originating from peripheral organs, such as adipose tissue and the gastrointestinal tract [2] . Leptin is a canonical weight-regulatory hormone that transduces adiposity signals to the hypothalamus [3] . By binding the long-form leptin receptor (LepRb) on hypothalamic neurons, leptin activates the Janus kinase 2—the signal transduction-activated transcript-3 (Stat3) signalling cascade [4] , [5] . Through this signalling pathway, leptin causes decreased energy intake and increased energy expenditure. In contrast to leptin, stomach-derived hormone ghrelin relays a hunger signal to the hypothalamus, which is partly achieved by counteracting hypothalamic leptin signalling [6] . Numerous hypothalamic intrinsic factors (melanocortins, Agouti -related protein, neuropeptide Y, melanin-concentrating hormone, endocannabinoids, serotonin, and so on) also have an important role in central regulation of energy metabolism [2] , [5] . Leptin and ghrelin exert their hypothalamic actions through modulation of these intrinsic factors [2] . Previous studies have demonstrated an involvement of apolipoproteins in hypothalamic appetite-regulatory pathways. Apolipoprotein AIV, D and E are produced in the hypothalamus and their expression levels are controlled by leptin [7] , [8] , [9] , [10] . Moreover, central administration of these apolipoproteins causes anorexia and weight loss in rodents [7] , [9] , [10] , indicating that hypothalamic apolipoproteins function as an intrinsic anorexigenic factor. However, the receptors and signalling pathways mediating these actions are entirely unknown. Clusterin, also known as apolipoprotein J (Apo-J), is a sulphated glycoprotein that is widely distributed in tissues, body fluids and fluid–tissue interfaces [11] , [12] . Clusterin has been implicated in a number of biological processes, such as immune modulation, sperm maturation, lipid transportation, neurodegeneration and cancer cell survival [13] , [14] , [15] , [16] , [17] . Interestingly, clusterin has been identified as a plasma leptin-binding partner and has been shown to modulate leptin signalling in LepRb-expressing cell lines [18] . Moreover, clusterin mRNA is highly expressed in the hypothalamic areas [19] that have a central role in the regulation of body weight and energy metabolism. However, no data are available about clusterin action on hypothalamic control of energy metabolism. LRP2 (low-density lipoprotein receptor-related protein-2, also called glycoprotein 330/megalin) is a multiligand endocytic receptor that belongs to the LRP family proteins [20] . LRP2 binds leptin to mediate leptin reuptake in renal tubules and to promote leptin transport across the choroid plexus [21] , [22] , [23] , suggesting a molecular link between LRP2 and leptin. LRP2 was also identified as an endocytic receptor for clusterin [24] , [25] and our preliminary data confirmed the mRNA expression of LRP2 in rodent hypothalamus. In this study we investigated the potential roles for hypothalamic clusterin and LRP2 in the regulation of energy homeostasis. Here we demonstrate clusterin and LRP2 are critical nodes in hypothalamic control of energy metabolism and may offer a novel target for the treatment of obesity-related metabolic diseases. Anorexigenic action of secretory clusterin Clusterin exists as two isoforms: a long (70–80 kDa) secretory isoform [11] and a short (~45 kDa) nuclear isoform [26] . To investigate the effect of clusterin on food intake and body weight we prepared a recombinant form of human secretory clusterin, which was disulphide-linked and glycosylated, similar to endogenous human plasma clusterin ( Supplementary Fig. S1 ). When administered into the third cerebroventricle adjacent to the hypothalamus, clusterin caused potent and prolonged inhibition of fasting-induced hyperphagia and weight gain ( Fig. 1a ). Pretreatment by intracerebroventricular (ICV) injection of clusterin suppressed hyperphagia induced by orexigenic neuropeptide Y (NPY) and Agouti -related peptide (AgRP) in freely fed mice ( Fig. 1b ). Consistently, continuous ICV infusion of clusterin (2 μg per day) using an osmotic pump resulted in chronic reduction of food intake, body weight and epididymal fat mass ( Fig. 1c ). In contrast, continuous ICV infusion of a neutralizing anticlusterin antibody increased food intake and body weight ( Fig. 1d ), suggesting that endogenous clusterin may exert anorexigenic and weight-reducing effects by acting in the hypothalamus. 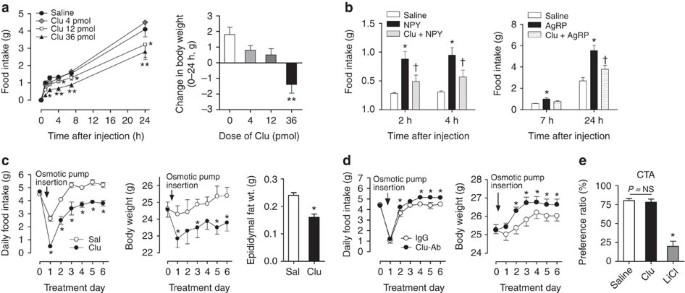Figure 1: Anorexigenic effects of secretory clusterin. (a) Effects of ICV administration of clusterin on food intake and body weight in overnight-fasted mice (n=6–7). *P<0.05, **P<0.01 versus saline. (b) Pretreatment with ICV administration of clusterin (1 μg) blocked NPY (1 μg)- and AgRP (4 μg)-induced hyperphagia in freely fed mice (n=6–7). *P<0.01 versus saline;†P<0.05 versus NPY or AgRP alone. (c) Continuous ICV infusion of clusterin (2 μg per day) via osmotic pump decreased food intake, body weight and visceral fat mass in mice (n=5). *P<0.05 versus saline on each treatment day. (d) Effects of ICV infusion of an anticlusterin neutralizing antibody (2 μg per day;n=5). *P<0.05 versus IgG on each treatment day. (e) The i.p. injection of lithium chloride but not ICV administration of clusterin induced CTA in mice (n=6–7). *P<0.01 versus saline. Statistical significance among the groups was tested using one-way analysis of variance (ANOVA) followed by apost-hocleast significant difference test (a,b,e). Statistical tests for chronic studies were conducted using repeated ANOVA (c,d). Data represent means±s.e.m. Figure 1: Anorexigenic effects of secretory clusterin. ( a ) Effects of ICV administration of clusterin on food intake and body weight in overnight-fasted mice ( n =6–7). * P <0.05, ** P <0.01 versus saline. ( b ) Pretreatment with ICV administration of clusterin (1 μg) blocked NPY (1 μg)- and AgRP (4 μg)-induced hyperphagia in freely fed mice ( n =6–7). * P <0.01 versus saline; † P <0.05 versus NPY or AgRP alone. ( c ) Continuous ICV infusion of clusterin (2 μg per day) via osmotic pump decreased food intake, body weight and visceral fat mass in mice ( n =5). * P <0.05 versus saline on each treatment day. ( d ) Effects of ICV infusion of an anticlusterin neutralizing antibody (2 μg per day; n =5). * P <0.05 versus IgG on each treatment day. ( e ) The i.p. injection of lithium chloride but not ICV administration of clusterin induced CTA in mice ( n =6–7). * P <0.01 versus saline. Statistical significance among the groups was tested using one-way analysis of variance (ANOVA) followed by a post-hoc least significant difference test ( a , b , e ). Statistical tests for chronic studies were conducted using repeated ANOVA ( c , d ). Data represent means±s.e.m. Full size image To exclude the possibility that clusterin-induced anorexia may be caused by general adverse effects or systemic toxicity, mice were subjected to a conditioned taste aversion (CTA) test. In contrast to intraperitoneal (i.p.) injection of lithium chloride, a well-known CTA inducer, which decreased saccharine consumption, ICV injection of clusterin had no effect on saccharine consumption, which indicated that clusterin did not induce CTA ( Fig. 1e ). Post brain-injury neuronal death is reduced in clusterin-deficient mice [16] ; thus, we tested whether ICV clusterin injection resulted in neuronal cell death in the hypothalamus. Clusterin treatment did not increase cell apoptosis in the hypothalamic area ( Supplementary Fig. S2 ), indicating that clusterin-induced anorexia and weight loss were unlikely due to neuronal cell death in the hypothalamus. Metabolic effect of altered hypothalamic clusterin expression We next investigated whether modulation of hypothalamic clusterin expression alters food intake and body weight. To increase hypothalamic clusterin expression, we administered adenoviruses expressing rat clusterin–green fluorescent protein (GFP) recombinant protein (Clu-Ad, 1 μl of 1 × 10 11 plaque-forming unit (p.f.u.)) into the bilateral mediobasal hypothalamus. We also injected the same amount of adenoviruses expressing GFP as a control and confirmed the proper injection of adenoviruses by examining GFP expression in the hypothalamus at the end of the study ( Supplementary Fig. S3 ). About 30~35% of the animals were excluded from the data analysis because of failure to target the mediobasal hypothalamus. Increased hypothalamic clusterin expression resulted in a decrease in food intake, body weight and abdominal fat mass ( Fig. 2a–c and Supplementary Fig. S4a ). 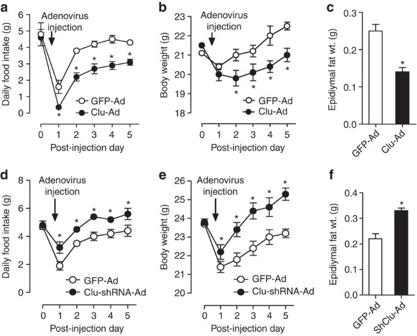Figure 2: Effects of altered hypothalamic clusterin. (a–c) Reduced food intake, body weight and epididymal fat weight in mice injected with a clusterin-expressing adenovirus (Clu-Ad) in bilateral mediobasal hypothalamus (n=5−6). (d–f) Increased food intake, body weight and intraabdominal fat mass in mice that received intrahypothalamic injection of an adenovirus expressing a clusterin-specific shRNA (Clu-shRNA-Ad) (n=5). *P<0.05 versus adenoviruses expressing GFP (GFP-Ad) on each treatment day. Statistical difference was tested using repeated analysis of variance (a,b,d,e) or an unpaired Student’st-test (c,f). Data represent means±s.e.m. Figure 2: Effects of altered hypothalamic clusterin. ( a – c ) Reduced food intake, body weight and epididymal fat weight in mice injected with a clusterin-expressing adenovirus (Clu-Ad) in bilateral mediobasal hypothalamus ( n =5−6). ( d – f ) Increased food intake, body weight and intraabdominal fat mass in mice that received intrahypothalamic injection of an adenovirus expressing a clusterin-specific shRNA (Clu-shRNA-Ad) ( n =5). * P <0.05 versus adenoviruses expressing GFP (GFP-Ad) on each treatment day. Statistical difference was tested using repeated analysis of variance ( a , b , d , e ) or an unpaired Student’s t -test ( c , f ). Data represent means±s.e.m. Full size image To suppress hypothalamic clusterin expression, we generated adenoviruses that expressed small-hairpin RNA specific to mouse clusterin(Clu-shRNA-Ad). Bilateral injection of Clu-shRNA-Ad into the mediobasal hypothalamus decreased clusterin expression by ~70% ( Supplementary Fig. S4b ). In these mice, food intake, body weight and abdominal fat weight were higher than those in mice injected with the same dose of adenoviruses expressing GFP ( Fig. 2d–f ). Taken together, these findings indicate that changes in hypothalamic clusterin expression could lead to altered body weight homeostasis. Metabolic regulation of hypothalamic clusterin expression Given the current evidence for an involvement of endogenous clusterin in hypothalamic control of energy balance, we examined clusterin expression levels under different feeding conditions or in response to metabolic hormones. In normal rats, food deprivation for 6–24 h resulted in a significant decrease in hypothalamic clusterin protein levels, whereas reestablishment of food intake after a 24-h fast correlated with an increase in hypothalamic clusterin protein ( Fig. 3a ), suggesting that increased hypothalamic clusterin in a postprandial state may contribute to the generation of satiety. Interestingly, the opposite dynamic was observed for clusterin concentrations in plasma and cerebrospinal fluid (CSF) in response to feeding/fasting ( Fig. 3a ). Similar to food intake, ICV administration of leptin (1 μg) in 24-h-fasted mice increased hypothalamic clusterin protein levels ( Fig. 3c ). In contrast, enhanced hypothalamic clusterin expression in a satiated condition was significantly decreased by ICV injection of the orexigenic hormone ghrelin (2 μg; Fig. 3d ), suggesting that hypothalamic clusterin expression levels are under the control of peripheral appetite-regulating hormones. 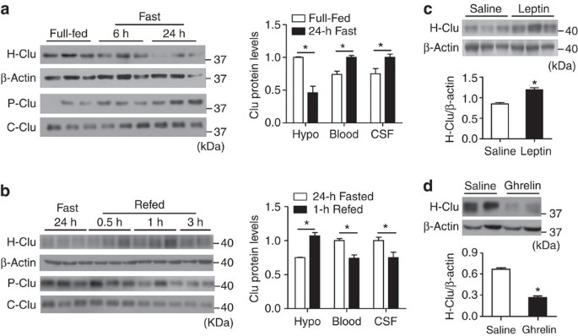Figure 3: Metabolic changes affect hypothalamic clusterin expression. (a) The effects of starvation on clusterin protein levels in the hypothalamus (H), plasma (P) and CSF (C) in satiated Sprague–Dawley rats (n=6). *P<0.05 versus full-fed group. (b) The effects of feeding on clusterin protein levels in the hypothalamus, plasma and CSF in 24-h-fasted Sprague–Dawley rats (n=6). *P<0.05 versus 24-h fasted group. (c) ICV administration of leptin in 24-h-fasted mice increased hypothalamic clusterin protein levels (n=5). *P<0.01 versus saline. (d) ICV administration of ghrelin to satiated mice decreased hypothalamic clusterin protein levels (n=5). *P<0.01 versus saline. Statistical significance was tested by an unpaired Student’st-test. Data represent means±s.e.m. Figure 3: Metabolic changes affect hypothalamic clusterin expression. ( a ) The effects of starvation on clusterin protein levels in the hypothalamus (H), plasma (P) and CSF (C) in satiated Sprague–Dawley rats ( n =6). * P <0.05 versus full-fed group. ( b ) The effects of feeding on clusterin protein levels in the hypothalamus, plasma and CSF in 24-h-fasted Sprague–Dawley rats ( n =6). * P <0.05 versus 24-h fasted group. ( c ) ICV administration of leptin in 24-h-fasted mice increased hypothalamic clusterin protein levels ( n =5). * P <0.01 versus saline. ( d ) ICV administration of ghrelin to satiated mice decreased hypothalamic clusterin protein levels ( n =5). * P <0.01 versus saline. Statistical significance was tested by an unpaired Student’s t -test. Data represent means±s.e.m. Full size image Clusterin activates hypothalamic Stat3 signalling Clusterin–leptin complexes activate Stat3 signalling in vitro [18] . To elucidate the signalling pathway involved in transduction of clusterin signals in the hypothalamus, immunohistochemical analysis of activated tyrosine (Tyr 705 )-phosphorylated Stat3 (phospho-Stat3) in the hypothalamus of mice was performed 30 min after ICV injection of leptin or clusterin (1 μg each). In agreement with previous reports [4] , ICV injection of leptin stimulated phospho-Stat3 expression in multiple areas of the hypothalamus, including the arcuate nucleus (ARC) and ventromedial nucleus ( Fig. 4a ). By comparison, ICV injection of clusterin resulted in strong Stat3 activation that was confined to the hypothalamic ARC ( Fig. 4a ). Double immunohistochemical staining for phospho-Stat3 and proopiomelanocortin (POMC) showed that similar to leptin, clusterin activated Stat3 signalling in POMC neurons ( Fig. 4c ). Dual assessment of fluorescence in situ hybridization (FISH) analysis of LepRb expression, followed with assessment of phospho-Stat3 by fluorescence immunohistochemistry, revealed that ICV administration of clusterin induced Stat3 activation in LepRb-expressing hypothalamic neurons, similar to leptin ( Fig. 4c ). The ability of clusterin to induce hypothalamic Stat3 activation was completely blocked by prior administration of its neutralizing antibody ( Fig. 4d ), suggesting that clusterin-induced Stat3 activation was not due to non-specific effects. 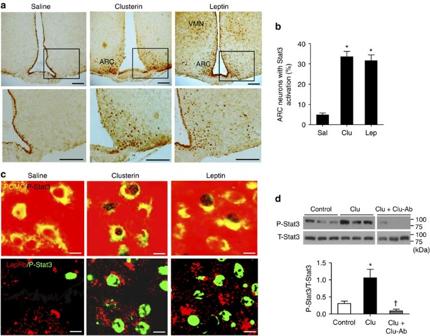Figure 4: Hypothalamic Stat3 activation by clusterin. (a,b) Immunohistochemical analysis of phospho-Stat3 (P-Stat3) in the hypothalamus 30 min after ICV administration of clusterin and leptin (n=3−4). ARC, arcuate nucleus; VMN, ventromedial nucleus; *P<0.01 versus saline. Scale bar, 200 μm. (c) Double immunostaining of phospho-Stat3 and POMC or LepRb in the hypothalamus 30 min after ICV administration of clusterin and leptin (n=3−4). Similar to leptin, clusterin increased nuclear localization of phospho-Stat3 in POMC- or LepRb-expressing hypothalamic neurons. Scale bar, 10 μm. (d) Pretreatment by ICV administration of anticlusterin neutralizing antibody (Clu-Ab: 1 μg) inhibited clusterin (1 μg)-induced hypothalamic Stat3 activation (n=3). *P<0.01 versus control;†P<0.01 versus clusterin alone. Statistical significance among the groups was tested using one-way analysis of variance followed by apost-hocleast significant difference. Data represent means±s.e.m. Figure 4: Hypothalamic Stat3 activation by clusterin. ( a , b ) Immunohistochemical analysis of phospho-Stat3 (P-Stat3) in the hypothalamus 30 min after ICV administration of clusterin and leptin ( n =3−4). ARC, arcuate nucleus; VMN, ventromedial nucleus; * P <0.01 versus saline. Scale bar, 200 μm. ( c ) Double immunostaining of phospho-Stat3 and POMC or LepRb in the hypothalamus 30 min after ICV administration of clusterin and leptin ( n =3−4). Similar to leptin, clusterin increased nuclear localization of phospho-Stat3 in POMC- or LepRb-expressing hypothalamic neurons. Scale bar, 10 μm. ( d ) Pretreatment by ICV administration of anticlusterin neutralizing antibody (Clu-Ab: 1 μg) inhibited clusterin (1 μg)-induced hypothalamic Stat3 activation ( n =3). * P <0.01 versus control; † P <0.01 versus clusterin alone. Statistical significance among the groups was tested using one-way analysis of variance followed by a post-hoc least significant difference. Data represent means±s.e.m. Full size image Hypothalamic LRP2 mediates metabolic effects of clusterin Previous studies have shown that clusterin binds to LRP2 (refs 24 , 25 ). As LRP2 was expressed in the mouse hypothalamus and SH-SY5Y neuronal cells ( Supplementary Fig. S5 ), we hypothesized that neuronal LRP2 may function as a receptor of clusterin in feeding regulation. The specific binding affinity (Kd) of clusterin to SH-SY5Y cells was 3.0 × 10 −10 M ( Supplementary Fig. S6 ). Clusterin binding was profoundly decreased when endogenous LRP2 expression was inhibited, suggesting that LRP2 mediates clusterin binding in these neuronal cells. Receptor-associated protein (RAP) inhibits the binding of ligands to LRP family proteins [27] . To investigate whether the hypothalamic actions of clusterin were mediated by LRP family proteins, RAP (3 μg) was administered into the cerebroventricle of overnight-fasted mice 30 min before injection of clusterin (1 μg). ICV injection of RAP alone did not significantly alter food intake. However, pretreatment with RAP inhibited the effects of exogenous clusterin on food intake and body weight by more than 80% when measured 24 h post injection ( Fig. 5a ). This inhibitory effect of RAP was sustained at 48 h post injection. Pretreatment with RAP also attenuated hypothalamic Stat3 activation induced by ICV injection of clusterin ( Fig. 5c ). To confirm that this inhibitory effect was specific for LRP2, a small interfering RNA specific to murine LRP2 (1 μmol; Dharmacon) was injected bilaterally into the mediobasal hypothalamus. Reduction of hypothalamic LRP2 expression significantly blunted the effects of ICV injection of clusterin (1 μg) on food intake and Stat3 activation ( Fig. 5d and Supplementary Fig. S7a ). These findings support a critical role for LRP2 in mediating the hypothalamic action of clusterin. As a recent study has demonstrated an involvement of hypothalamic LRP1 in central leptin signalling and body weight homeostasis [28] , we examined the effects of LRP1 inhibition on clusterin-mediated regulation of feeding behaviour. Hypothalamic LRP1 inhibition significantly impaired clusterin-induced anorexia and Stat3 activation ( Supplementary Figs S7b and S8 ). These results indicated that both LRP1 and LRP2 may have similar functions in hypothalamic clusterin signalling. 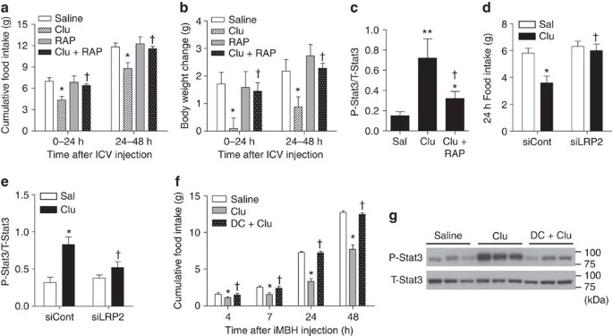Figure 5: Hypothalamic LRP2 mediates the effects of clusterin. (a–c) Pretreatment with ICV administration of RAP inhibited clusterin-induced anorexia, weight loss and hypothalamic Stat3 activation (n=6–7). *P<0.05, **P<0.01 versus saline;†P<0.05 versus clusterin alone. (d,e) The effects of clusterin on food intake and hypothalamic Stat3 phosphorylation were attenuated in mice injected with LRP2 siRNA (siLRP2) (n=5–6). *P<0.05 versus control siRNA (siControl) and saline groups;†P<0.05 versus siControl and clusterin groups. (f,g) Prior intrahypothalamic administration of dansylcadaverine (DC), a clathrin-dependent endocytosis inhibitor, inhibited clusterin (0.1 μg)-induced anorexia and Stat3 activation (n=6−7). *P<0.05 versus saline;†P<0.05 versus clusterin alone. Statistical significance among the groups was tested using one-way ANOVA (a–c,f,g) or a two-way analysis of variance (d,e). Data represent means±s.e.m. Figure 5: Hypothalamic LRP2 mediates the effects of clusterin. ( a – c ) Pretreatment with ICV administration of RAP inhibited clusterin-induced anorexia, weight loss and hypothalamic Stat3 activation ( n =6–7). * P <0.05, ** P <0.01 versus saline; † P <0.05 versus clusterin alone. ( d , e ) The effects of clusterin on food intake and hypothalamic Stat3 phosphorylation were attenuated in mice injected with LRP2 siRNA (siLRP2) ( n =5–6). * P <0.05 versus control siRNA (siControl) and saline groups; † P <0.05 versus siControl and clusterin groups. ( f , g ) Prior intrahypothalamic administration of dansylcadaverine (DC), a clathrin-dependent endocytosis inhibitor, inhibited clusterin (0.1 μg)-induced anorexia and Stat3 activation ( n =6−7). * P <0.05 versus saline; † P <0.05 versus clusterin alone. Statistical significance among the groups was tested using one-way ANOVA ( a – c , f , g ) or a two-way analysis of variance ( d , e ). Data represent means±s.e.m. Full size image The LRP family proteins have been identified as endocytic receptors [20] , [24] . Traditionally, endocytosis has been viewed as a mechanism for receptor downregulation, thereby desensitizing cells to signalling molecules. However, recent work has shown that endocytosis is also an essential process in signal transduction by hormones, growth factors and other cell modulators [29] . Intrahypothalamic injection of the clathrin-dependent endocytosis inhibitor dansylcadaverine (25 pmol) attenuated anorexia and Stat3 phosphorylation in response to clusterin (0.5 μg; Fig. 5f ). These findings suggested that endocytosis may be a pivotal step during the course of clusterin-induced anorexia and Stat3 activation in the hypothalamus. Clusterin induces interactions of LRP2 and LepRb A recent paper demonstrated a direct interaction between LRP1 and LepRb (ref. 28 ). We therefore studied the in vivo dynamics of LepRb and LRP2 in response to clusterin treatment by using fluorescence cross-correlation spectroscopy [30] , wherein interaction strength was measured as a cross-correlation function [G(τ)]. In primary cultures of human neuronal cells transiently transfected with expression vectors for fluorescent fusion proteins of LepRb (LepRb–EGFP) and LRP2 (LRP2–tagRFP), treatment with clusterin (1 nM) significantly increased the cross-correlation coefficient for EGFP and tagRFP compared with the saline-treated control, suggesting that LRP2 and LepRb physically interact upon binding to clusterin ( Fig. 6a ). These data were further confirmed by a proximity ligation assay showing that clusterin could rapidly induce the colocalization of LepRb and LRP2 ( Fig. 6b ). These findings raised the question as to whether LepRb could be involved in hypothalamic clusterin signalling pathway. In LepRb-deficient db/db mice, the effects of clusterin to decrease food intake and body weight, and to increase Stat3 phosphorylation were abolished ( Fig. 6c–e ), indicating that LepRb is required for clusterin action and signalling. 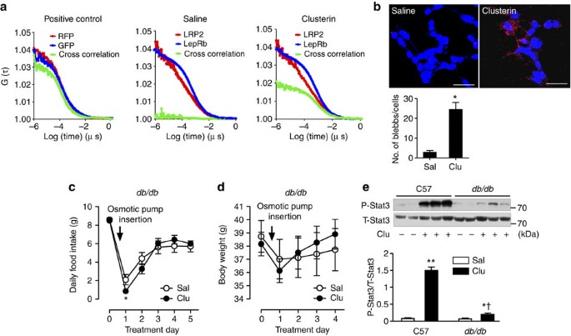Figure 6: Clusterin-induced interaction between LRP2 and LepRb. (a) The interaction dynamics between LepRb and LRP2 following clusterin treatment was assessed by fluorescence cross-correlation spectroscopy (FCCS) in primary cultured human neurons. Inxaxis: log lag time during measurement; inyaxis: autocorrelation and cross-correlation (CC) function [G(τ)]. CC indicates the strength of the physical interaction between LepRb and LRP2. Data represent the average values of ten measurements. (b) Proximity ligation assay of the interaction (red spots, blobs) between LepRb and LRP2 upon clusterin treatment in primary cultured human neurons. Nuclei were visualized by Hoechst 33342 staining (blue). Scale bar, 25 μm. *P<0.005 versus saline. (c,d) Effects of chronic ICV infusion of clusterin (2 μg per day) on food intake and body weight indb/dbmice. *P<0.05 versus saline. (e) Impaired hypothalamic Stat3 activation in response to ICV injection of clusterin (1 μg) indb/dbmice (n=4−5). *P<0.05, **P<0.005 versus saline in each mouse group;†P<0.005 versus clusterin-treated C57 mice. Statistical significance among the groups was tested using an unpaired Student’st-test (b), repeated analysis of variance (ANOVA) (c,d) or two-way ANOVA (e). Data represent means±s.e.m. Figure 6: Clusterin-induced interaction between LRP2 and LepRb. ( a ) The interaction dynamics between LepRb and LRP2 following clusterin treatment was assessed by fluorescence cross-correlation spectroscopy (FCCS) in primary cultured human neurons. In x axis: log lag time during measurement; in y axis: autocorrelation and cross-correlation (CC) function [G(τ)]. CC indicates the strength of the physical interaction between LepRb and LRP2. Data represent the average values of ten measurements. ( b ) Proximity ligation assay of the interaction (red spots, blobs) between LepRb and LRP2 upon clusterin treatment in primary cultured human neurons. Nuclei were visualized by Hoechst 33342 staining (blue). Scale bar, 25 μm. * P <0.005 versus saline. ( c , d ) Effects of chronic ICV infusion of clusterin (2 μg per day) on food intake and body weight in db/db mice. * P <0.05 versus saline. ( e ) Impaired hypothalamic Stat3 activation in response to ICV injection of clusterin (1 μg) in db/db mice ( n =4−5). * P <0.05, ** P <0.005 versus saline in each mouse group; † P <0.005 versus clusterin-treated C57 mice. Statistical significance among the groups was tested using an unpaired Student’s t -test ( b ), repeated analysis of variance (ANOVA) ( c , d ) or two-way ANOVA ( e ). Data represent means±s.e.m. Full size image Hypothalamic clusterin expression and action in obesity A defect in the ability to generate appropriate satiety signals in the hypothalamus is believed to be a major cause of obesity in humans and animals. We further tested the possibility that dysregulation of hypothalamic clusterin may contribute to defective satiety signalling in obese mice. Unlike lean mice, diet-induced obese (DIO) mice displayed no sizable change in hypothalamic clusterin expression in response to food intake or leptin ( Fig. 7a ). In these DIO mice, repeated ICV injection of clusterin (1 μg per day) caused a significant reduction in food intake, body weight and fasting blood glucose ( Fig. 7c–e ). These data suggest that the inability to increase anorexigenic clusterin in the hypothalamus may lead to overeating in the obese condition and further implicate that treatment with clusterin supplementation may provide significant benefits in obese individuals. 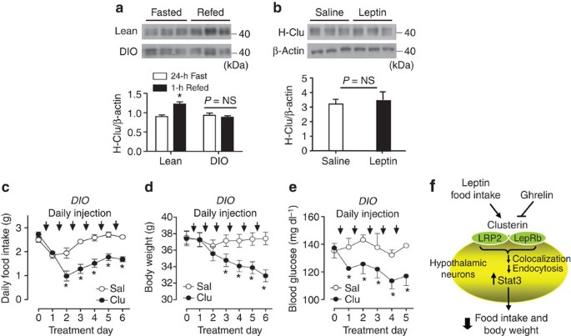Figure 7: Dysregulated hypothalamic clusterin in DIO mice and antiobesity effects of clusterin. (a,b) Feeding- and ICV leptin-induced increases in hypothalamic clusterin levels were abolished in DIO mice (n=6). Analysis of hypothalamic clusterin expression was performed in 24-h fasting and 1-h refeeding condition, or 1 h after ICV injection of saline and leptin. *P<0.05 versus fasted lean mice. NS, not significant. (c–e) Effect of repeated ICV injection of clusterin on food intake, body weight and plasma glucose concentrations in DIO mice (n=6). *P<0.05 versus saline on each treatment day. Statistical significance among the groups was tested using an unpaired Student’st-test (a,b) or repeated analysis of variance (c,d,e). (f) Schematic representation of the proposed role of hypothalamic clusterin and LRP2 in the feeding regulatory circuit. Figure 7: Dysregulated hypothalamic clusterin in DIO mice and antiobesity effects of clusterin. ( a , b ) Feeding- and ICV leptin-induced increases in hypothalamic clusterin levels were abolished in DIO mice ( n =6). Analysis of hypothalamic clusterin expression was performed in 24-h fasting and 1-h refeeding condition, or 1 h after ICV injection of saline and leptin. * P <0.05 versus fasted lean mice. NS, not significant. ( c – e ) Effect of repeated ICV injection of clusterin on food intake, body weight and plasma glucose concentrations in DIO mice ( n =6). * P <0.05 versus saline on each treatment day. Statistical significance among the groups was tested using an unpaired Student’s t -test ( a , b ) or repeated analysis of variance ( c , d , e ). ( f ) Schematic representation of the proposed role of hypothalamic clusterin and LRP2 in the feeding regulatory circuit. Full size image The current study provides new evidence of a physiological role of clusterin in the hypothalamic regulation of energy balance. Central administration of clusterin suppressed fasting-, NPY- and AgRP-induced feeding and weight gain, whereas inhibition of hypothalamic clusterin action promoted food intake and weight gain. Furthermore, hypothalamic clusterin levels were greatly increased by the satiety hormone leptin, but deceased by the hunger hormone ghrelin, suggesting that endogenous hypothalamic clusterin may serve as a novel anorexigenic molecule. Our data demonstrate that clusterin activated Stat3 signalling in hypothalamic neurons, including POMC- and LepRb-expressing neurons, raising the possibility that clusterin signalling could be related to leptin signalling. Indeed, we found that treatment of cultured neuron cells with clusterin rapidly induced the physical interaction of functional leptin receptor LepRb and LRP2. Moreover, clusterin-induced anorexia and hypothalamic Stat3 activation were dependent on LepRb and LRP2. Along with this, it has been reported that LRP1 forms the molecular complex with leptin–LepRb in hypothalamic neurons, and neuronal deletion of LRP1 results in leptin resistance and obesity [28] . Collectively, these findings indicate a significant role for LRP family proteins in hypothalamic leptin and clusterin signalling. It is evident that in addition to clusterin (Apo-J), other types of apolipoprotein are involved in hypothalamic control of energy homeostasis. Apolipoprotein E is expressed in hypothalamic astrocytes and neurons [10] . Expression of Apo-AIV, known as a gastrointestinal satiety protein, is also found in hypothalamic neurons [7] , [8] . Apolipoprotein D, a lipocalin highly expressed in the brain, is coexpressed with LepRb in hypothalamic neurons [9] . Hypothalamic expression levels of these apolipoproteins are increased by leptin administration and reduced in several mice models of obesity [7] , [9] , [10] . Furthermore, ICV administration of those apolipoproteins induces a significant anorexia [7] , [9] , [10] . Despite apparent appetite-regulating effects of these apolipoproteins, their receptors and signalling pathways in the hypothalamus remain elusive. Given that clusterin (Apo-J) regulates food intake via LRP2, it will be important to test if other apolipoproteins may regulate feeding behaviour through LRP2 and other LRP family proteins. Clusterin is highly expressed in the central nervous system and in systemic circulation [19] , [31] . Notably, food ingestion induced reciprocal changes in central and peripheral clusterin expression, that is, increased levels in the hypothalamus, but decreased levels in plasma and CSF. Feeding-related changes in hypothalamic clusterin levels fit well with its anorexigenic effects. Consistently, we found that manipulation of clusterin expression in the hypothalamus altered food intake and body weight. As 125 I-Apo-AIV was barely detectable in the brain when systemically administered [8] , it is conceivable that most of hypothalamic apolipoproteins may be synthesized in the brain. These data support a critical role for brain-derived apolipoproteins, including clusterin, in the context of energy homeostasis. Interestingly, clusterin specifically stimulated Stat3 phosphorylation in the mediobasal hypothalamus. Clusterin expression levels in this area were increased by leptin, but this response was abolished in DIO mice. It is therefore likely that failure to increase hypothalamic clusterin in response to leptin may confer impaired Stat3 activation in the mediobasal hypothalamus of obese mice, which is a key feature of obesity-associated central leptin resistance [32] . This study also revealed that supplement of clusterin in leptin-resistant obese mice was able to suppress food intake and weight gain, indicating that clusterin can be used to treat central leptin resistance and obesity. However, it was noted that chronic treatment of clusterin caused a modest decrease in food intake and body weight. The reason for this is unclear at this time. Chronic elevation of clusterin levels by continuous infusion in the hypothalamic extracellular fluid may induce internalization of clusterin–LRP2 complexes in hypothalamic neurons, resulting in reduced LRP2 expression on the plasma membrane and desensitization of hypothalamic neurons to exogenous clusterin. It is also possible that chronic administration of clusterin activates negative feedback signalling pathways or as yet unidentified neuronal population that counteracts anorexigenic effects of clusterin. Thus, the validity of antiobesity treatment using clusterin needs to be further tested. From the results of the current study, we propose a new model of the hypothalamic feeding regulatory circuit ( Fig. 7f ). Hypothalamic clusterin contents are increased during the postprandial period. Clusterin interacts with LRP2 and LepRb on the plasma membrane of hypothalamic neurons, leading to colocalization of LepRb and LRP2. This ligand–receptor complex may be subjected to endocytosis and may interact with signalling molecules, such as Stat3, to further activate downstream signalling. As a result, clusterin may generate a satiety signal in hypothalamic neurons. Emergence of clusterin and LRP2 as novel appetite regulators could lead to new therapeutic options for obese individuals with leptin resistance. Synthesis of secretory clusterin A complementary DNA for the secretory isoform of human clusterin was amplified from a commercially obtained human transcriptome (Stratagene, CA) using the following primers: 5′-gcgcaagcttggaggcatgatgaagactctgct-3′ and 5′-gcgcgtcgaccaccacccggtgctttttgcggta-3′. The amplified fragment was cloned into pAGCF and then the vector was transfected into HEK293 cells. Serum-free culture supernatants were collected, concentrated by ultrafiltration and then applied to an anti-FLAG (M2) column (Sigma). Recombinant secretory clusterin (AdipoGen AG-40A-0050; Incheon, Korea) was eluted with buffer containing FLAG peptide (DYKDDDDK) and then dialysed against PBS. Cell culture SH-SY5Y neuroblastoma cells (ATCC, CRL-2266) were maintained in DMEM containing 10% FCS, penicillin and streptomycin (100 units per ml each). Human brain tissue used for primary cultures of human neuronal cells was obtained from the Brain Bank of Seoul National University Hospital (Seoul, Korea). Animals Male C57BL/6 mice and Sprague–Dawley rats, 8–12 weeks of age were obtained from Orient Bio (Seoul, Korea). The male db/db mice were purchased from SLC (Hamamatsu, Japan). Animals were fed a standard chow diet (Samyang, Seoul, Korea) ad libitum , unless otherwise indicated, housed in a controlled temperature environment (22±1 °C) and subjected to a 12 h light–dark cycle (light from 0700 to 1900, h). DIO mice were obtained by feeding mice a high-fat diet (60% fat; Research Diet Co., New Brunswick, NJ) for 8–10 weeks. Lean controls were fed a low-fat diet (10% fat) for the same period. Plasma glucose concentrations were measured using a glucose analyser (YSI 2300, Yellow Springs, OH). All of the animal procedures were approved by the Institutional Animal Care and Use Committee of the Asan Institute for Life Sciences (Seoul, Korea). Cannulation and injection Permanent 26-gauge stainless steel cannulae were implanted into the third ventricle (1.8 mm caudal to bregma and 5.0 mm ventral to the sagittal sinus) or into the mediobasal hypothalamus (1.8 mm caudal to bregma, 0.25 mm lateral and 5.5 mm ventral to the sagittal sinus) of mice. After a 1-week recovery period, mice were handled daily for 3 days to acclimatize them to the injection procedure. Clusterin, leptin, ghrelin (Phoenix Pharmaceuticals, Belmont, CA), RAP (Molecular Innovations, Southfield, MI), dissolved in 0.9% (w/v) saline and dansylcadaverine (Sigma), dissolved in 10% dimethylsulphoxide, were administered in a total volume of 3 μl for ICV injections and 1 μl for intrahypothalamic injections. To assess the feeding response to anticlusterin antibodies, mice received a continuous ICV infusion of anticlusterin–α/β antibody (2 μg per day; Santa Cruz, H-330) or anti-rabbit IgG (2 μg per day, Amersham) as a control, via an Alzet osmotic mini-pump placed subcutaneously in the interscapular area. Most experiments were performed early in the light phase (between 0900 and 1100, h) in overnight-fasted mice, unless indicated. NPY and AgRP (Phoenix Pharmaceuticals) were administered to mice that had free access to food. Food intake and body weight were monitored for 2 days post injection. Adenovirus and siRNA experiments Adenovirus vectors encoding GFP, recombinant clusterin or a clusterin-specific shRNA (target nucleotides 444–462) conjugated to GFP were purified by CsCl gradient centrifugation and filtered to a concentration of ~10 −11 p.f.u. ml −1 . Adenoviruses were injected into the bilateral ARC (5.7 mm depth, 1.8 mm caudal to bregma, 0.25 mm lateral from the sagittal suture) via a syringe pump (Harvard Apparatus, Holliston, MA) at a rate of 100 nl min −1 for 5 min (0.5 μl per injection site). Food intake and body weight were monitored daily after adenovirus injection, and then animals were killed on the fifth day after a 5-h fast. The brain and epididymal fat were collected. Correct injection of adenovirus was verified by monitoring green fluorescence in the hypothalamus by confocal microscopy at the end of the experiment. Only animals in which correct injection was confirmed were included in the analysis ( Supplementary Fig. S3 ). In a separate experiment, we determined hypothalamic clusterin expression using immunoblottings following adenovirus treatment. Injection of a clusterin-expressing adenovirus increased hypothalamic clusterin levels ~2.8-fold, whereas injection with a clusterin shRNA-expressing adenovirus decreased hypothalamic clusterin levels by 65% ( Supplementary Fig. S4 ). The siRNA particles targeting murine LRP2 and LRP1 (Dharmacon, Chicago, IL) were resuspended in RNase-free water, mixed with Lipofectamine (9:1 v/v; Invitrogen, Carlsbad, CA) to a final concentration of 1 mM, and were then injected bilaterally into the mediobasal hypothalamus (0.5 μl each side) as described above. The same amount of an untargeted scrambled control siRNA (Dharmacon) was administered to the control group. Gene knockdown was considered successful when hypothalamic LRP1 and LRP2 expression levels were less than 30% of the average expression level in the control group ( Supplementary Fig. S7 ). Only animals in which gene knockdown was confirmed were included in the data analysis. Conditioned taste aversion test Mice were habituated to 1 h daily access to water for 7 days. Immediately following the 1-h exposure of two bottles containing 0.15% saccharin, mice received sequential injections of i.p. saline followed by ICV saline, i.p. lithium chloride (127 mg kg −1 ; Sigma) followed by ICV saline, or i.p. saline followed by ICV clusterin (1 μg). For 3 consecutive days thereafter, a two-bottle choice test was conducted. The preference ratio was calculated as the intake of saccharine solution/total intake of water and saccharine solution. Immunoblot analysis Hypothalamic tissue lysates (30 μg protein) were subjected to immunoblot analysis using antibodies against the clusterin β-chain (1:1,000; Santa Cruz) or phospho- and total Stat3 (1:1,000; Cell Signaling). Rat plasma (diluted to 1:250) and non-diluted CSF were used for clusterin immunoblotting. Protein band density was quantitated using a densitometer (VersaDoc Multi Imaging Analyzer System; Bio-Rad). Results were normalized to β-actin (for clusterin) or total Stat3 (for phospho-Stat3). Please see Supplementary Fig. S9 for complete gel data. Immunohistochemistry and immunofluorescence staining Thirty minutes after ICV injection of leptin and clusterin, mice under anaesthesia were perfused through the heart with 10% formalin for 15 min, using a peristaltic pump. To verify Stat3 phosphorylation in the hypothalamus, hypothalamic tissue slices were incubated overnight with a rabbit anti-phospho-Stat3 antibody (1:100; Cell Signaling) at 4 °C. Tissue sections were rinsed with PBS and then incubated for 1 h at room temperature with goat anti-rabbit IgG (1:100; Vector Laboratories). Immunoreactive proteins were visualized by incubation with 3,3′-diaminobenzidine tetrahydrochloride in 0.1 M Tris-HCl buffer (pH 7.2). For double immunostaining of POMC and phospo-Stat3, tissue sections were first subjected to phospho-Stat3 immunostaining as described above and then incubated overnight at 4 °C with a rabbit anti-POMC antibody (1:150; Phoenix Pharmaceuticals). Tissues were rinsed with PBS and then incubated for 1 h at room temperature with Alexa Fluor 488-conjugated anti-rabbit IgG (1:500; Invitrogen). After washing with PBS, tissue slices were mounted using Vectashield mounting media (Vector Laboratories) and viewed using an LSM 700 confocal microscope (Carl Zeiss). Fluorescence in situ hybridization FISH analysis was performed using a FISH Tag RNA Red Kit with Alexa Fluor 594 dye (Invitrogen). RNA probes were prepared by in vitro transcription using a LepRb cDNA as a template, followed by denaturation for 2 min at 55 °C in hybridization buffer, after which the probes were kept on ice. Hypothalamic slices were incubated for 20 h at 55 °C with denatured fluorescent dye-labelled RNA. After sequential rinsing with hybridization buffer and PBS, tissues were incubated overnight at 4 °C with a rabbit anti-phospho-Stat3 antibody (1:100; Cell Signaling). Finally, tissue slices were rinsed with PBS and incubated for 1 h at room temperature with Alexa Fluor 488-conjugated anti-rabbit IgG (1:500). Fluorescence cross-correlation spectroscopy Fluorescence cross-correlation spectroscopy was used to measure the molecular interaction between LepRb and LRP2 (ref. 30 ). In brief, primary cultured human neurons were transfected with very low amounts (0.005 μg each) of LepRb–EGFP and/or LRP2–tagRFP by using Lipopectamine (Invitrogen) to minimize perturbation of the cells. Forty-eight hours after transfection, cells were serum-starved for 2 h and then treated with clusterin (1 nM) for 1 min. Fluorescence cross-correlation spectroscopy was performed in live neurons at 25 °C, using an inverted confocal laser scanning microscope (LSM710-ConfoCor3, Carl Zeiss). For each sample, the measurement was taken ten times for 15–20 s each time. Data were analysed using the ConfoCor3 software and represent average values. Proximity ligation assay To visualize the physical interaction between LepRb and LRP2, primary cultured human neurons were treated with clusterin (1 nM) for 1 min and then fixed with 100% methanol for 20 min at room temperature. Cells were incubated with a mouse anti-LepRb (1:100; Alpha Diagnostics, catalogue number OBR130A; San Antonio, TX) and rabbit anti-LRP2 (1:200; Santa Cruz) primary antibodies at 4 °C overnight. The proximity ligation assay (PLA) was performed using a Duolink in situ PLA kit (Olink Bioscience, Uppsala, Sweden) with PLA plus and minus probes for rabbit and mouse antiserum. Cell nuclei were visualized using Hoechst 33342 (Olink Bioscience). Specimens were examined by confocal microscopy. The number of in situ PLA signals per cell was counted by semiautomated image analysis using BlobFinder software (Olink Bioscience). For each experiment, three fields were measured and the data represent three independent experiments. Analysis of mRNA expression Total RNA was extracted using Trizol reagents (Invitrogen). The mRNA expression levels of clusterin, LepRb, LRP2, LRP1, VLDL-R and ApoER2 were determined by real-time PCR or semiquantitative reverse transcriptase–PCR using the primers listed in Supplementary Table S1 . The expression of each mRNA was normalized to that of glyceraldehyde 3-phosphate dehydrogenase. Statistical analysis Data represent means±s.e.m. Statistical analysis was performed using SPSS-PC14 (Chicago, IL). Statistical significance among the groups was tested using one-way or repeated analysis of variance, followed by a post-hoc least significant difference test or an unpaired Student’s t -test, when appropriate. A two-way analysis of variance was used to study the effects of ICV injection of clusterin in db/db mice and siRNAs. Statistical significance was defined as P <0.05. How to cite this article: Min-Seon, K. et al . Clusterin and LRP2 are critical components of the hypothalamic feeding regulatory pathway. Nat. Commun. 4:1862 doi: 10.1038/ncomms2896 (2013).